Tissue landscape alters adjacent cell fates duringDrosophilaegg development Extracellular signalling molecules control many biological processes, but the influence of tissue architecture on the local concentrations of these factors is unclear. Here we examine this issue in the Drosophila egg chamber, where two anterior cells secrete Unpaired (Upd) to activate Signal transducer and activator of transcription (STAT) signalling in the epithelium. High STAT signalling promotes cell motility. Genetic analysis shows that all cells near the Upd source can respond. However, using upright imaging, we show surprising asymmetries in STAT activation patterns, suggesting that some cells experience different Upd levels than predicted by their location. We develop a three-dimensional mathematical model to characterize the spatio–temporal distribution of the activator. Simulations show that irregular tissue domains can produce asymmetric distributions of Upd, consistent with results in vivo . Mutant analysis substantiates this idea. We conclude that cellular landscape can heavily influence the effect of diffusible activators and should be more widely considered. During animal development, cells must respond to a changing environment and adopt proper identities. Diffusible, extracellular signals often instruct cells to take on particular fates. A classic type of instructive signal, called a morphogen, acts to pattern tissues in a concentration-dependent manner. While tissues are developing, a morphogen released from a defined region (source) creates a concentration gradient as the protein diffuses, and either interacts with a target cell or decays. In target cells, the morphogen level determines the appropriate response: concentrations above a certain threshold elicit one response, whereas those over another threshold prompt a different response. Thus, each cell receives positional information based on the gradient and this determines its fate (reviewed in refs 1 , 2 , 3 ). Our understanding of diffusible activators such as morphogens comes from a variety of contexts, but most studies presuppose that these signalling molecules act within a uniform landscape. During animal development, however, signalling occurs between cells that are packed into complex shapes. To understand how the intricate architecture of tissues can influence diffusible signals and pattern generation, we have focused on the egg development of Drosophila melanogaster . The Drosophila egg chamber consists of germline and somatic cells, which are coordinated in their development. A single-layer epithelium of somatic follicle cells surrounds the oocyte and 15 large nurse cells that support egg growth [4] . Not all follicle cells are equivalent. Instead, multiple signalling pathways converge to define distinct subsets of cells (reviewed in refs 5 , 6 , 7 , 8 ). One early event is the specification of two pairs of specialized follicle cells, called polar cells, at the anterior and posterior poles of the epithelium. In mid-oogenesis, the two anterior polar cells secrete a ligand that specifies the nearest 6–8 follicle cells as a migratory cell type, the border cells [9] , [10] , [11] , [12] , [13] , [14] . Hours later, the border cells detach from the epithelium and migrate towards the oocyte, where they are required to make a viable egg, and remaining anterior follicle cells stretch over the nurse cells. Anterior polar cells instruct neighbouring cell fates by activating the well-conserved Janus tyrosine kinase (JAK), and Signal transducer and activator of transcription (STAT) pathway (reviewed in refs 5 , 15 , 16 , 17 ). Polar cells secrete a diffusible signal, Unpaired (Upd), which acts as a morphogen. The Upd glycoprotein associates with heparin sulfate proteoglycans along follicle cells, which helps to establish its graded distribution as observed in fixed tissues [14] , [18] . Upd binds to a transmembrane receptor, Domeless (Dome), on neighbouring cells, thereby inducing JAK-mediated phosphorylation of associated STAT molecules [5] , [9] , [10] , [11] , [16] . Phospho-STAT dimers move to the nucleus and activate transcription. One direct STAT target gene is slow border cells ( slbo ), which encodes a transcription factor required for border cell migration [10] , [11] , [12] , [13] . The gradient of Upd is reflected by the graded pattern of Slbo and STAT nuclear expression at the anterior pole; cells with the highest levels of these proteins become the motile border cells [12] , [19] . Although about 12 cells initially display STAT activation typically, only 6–8 maintain the above-threshold signalling needed for Slbo expression and border cell specification, whereas the other cells switch the signal off [19] , [20] . Mutations that disrupt STAT signalling result in too many or too few migratory cells and poor migration [9] , [10] , [11] , [21] , [22] . Thus, precise regulation of STAT activity ensures proper egg chamber development. One key STAT activity regulator in follicle cells is Apontic (Apt). Apt is widely expressed and serves as a feedback inhibitor of STAT signalling [19] , [20] , [23] . In loss-of-function apt mutants, anterior follicle cells activate STAT to a greater extent than normal, resulting in additional motile cells. Thus, Apt normally sets a high threshold for STAT-activated motility, and acts to shut off STAT function in cells with intermediate or low levels of activation. This genetic inhibition limits the number of motile cells specified in the anterior epithelium. Upd secreted apically by the polar cells diffuses beneath the epithelium [14] into an extracellular domain bounded by the neighbouring nurse cells. Because the nurse cells are very large, their membranes create an irregular region adjacent and subapical to the follicle cells ( Fig. 1a,b ). To investigate whether this landscape of neighbouring tissue influences morphogen-mediated cell fate decisions in the follicular epithelium, we developed a new strategy to view egg chambers [24] . This protocol positions the polar cells above the nurse cells, providing a unique perspective. If the contour of the adjacent germline cells did not alter morphogen signalling, we would anticipate uniform STAT activation around the polar cells when viewed upright; in contrast, asymmetry in cell fate patterning could suggest influence by the nurse cells or the irregular extracellular domain they create. 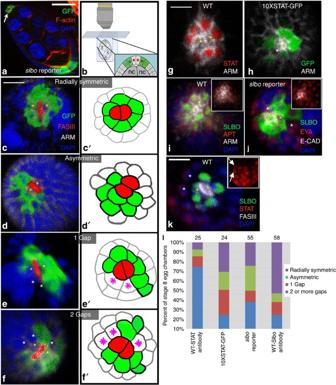Figure 1: Upright imaging reveals multiple patterns of STAT activation in follicular epithelia. (a) Lateral view of a stage 8slbo-reporter egg chamber; presumptive border cells are GFP positive (green, arrow), F-actin (phalloidin) is shown in red and nuclei (4,6-diamidino-2-phenylindole (DAPI)) are blue. Scale bar, 50 μm. (b) Schematic of upright egg chamber imaging technique. Inset shows presumptive border cells (green), polar cells (red nuclei), nurse cells (nc), and the extracellular subapical space between the epithelium and nurse cells (white). (c–k) Three-dimensional reconstructions of optical sections, projected into one plane, from the anterior epithelia of stage 8 egg chambers. Yellow asterisks mark polar cells. Scale bar, 10 μm. (c–f) Egg chambers fromslbo-reporter (GFP, green) flies. White asterisks mark ‘gap cells’: GFP-negative cells contacting the polar cells. Fasciclin III (Fas III) is red; Armadillo (Arm), white; DAPI, blue. See alsoSupplementary Fig. 1. (c′–f′) Schematics of cell organizations. Polar cells, red; presumptive border cells, green; gap cells, magenta asterisks. (c,c′) Radially symmetric organization ofslbo-positive cells. (d,d′) Asymmetric organization ofslbo-positive cells. (e,e′) One gap inslbo-positive cells around the polar cells. (f,f′) Two gaps in organization ofslbo-positive cells. (g) STAT expression (red) is radially symmetric around the polar cells in seven neighbouring cells in wild type (WT; Canton S). (Arm, white.) (h) STAT activity (green) shows one gap around the polar cells, indicated by lack of 10XSTAT-GFP expression (white asterisk). (Arm, white.) (i) Seven Slbo-expressing cells (green) radially symmetric around the polar cells (yellow asterisks) in wild type. Apt, red, inset; Arm, white; DAPI, blue. (j) Two gaps (white asterisks) inslbo-reporter activation (green) next to the polar cells (yellow asterisks). Eyes absent (Eya), red, inset; E-cadherin (E-CAD), white; DAPI, blue. (k) Slbo protein (green) present in cells to one side of polar cells (yellow asterisks) (Fas III, white) and absent from two cells (white asterisks), although STAT (red, inset, arrows) is detected. (l) Proportions of four classes of organization patterns in the first tier of cells contacting the polar cells using four different markers/genotypes (bottom). Forslboreporter and 10XSTAT-GFP, positive cells were scored by GFP antibody staining. Numbers of egg chambers scored (n) shown at the top. Figure 1: Upright imaging reveals multiple patterns of STAT activation in follicular epithelia. ( a ) Lateral view of a stage 8 slbo -reporter egg chamber; presumptive border cells are GFP positive (green, arrow), F-actin (phalloidin) is shown in red and nuclei (4,6-diamidino-2-phenylindole (DAPI)) are blue. Scale bar, 50 μm. ( b ) Schematic of upright egg chamber imaging technique. Inset shows presumptive border cells (green), polar cells (red nuclei), nurse cells (nc), and the extracellular subapical space between the epithelium and nurse cells (white). ( c–k ) Three-dimensional reconstructions of optical sections, projected into one plane, from the anterior epithelia of stage 8 egg chambers. Yellow asterisks mark polar cells. Scale bar, 10 μm. ( c–f ) Egg chambers from slbo -reporter (GFP, green) flies. White asterisks mark ‘gap cells’: GFP-negative cells contacting the polar cells. Fasciclin III (Fas III) is red; Armadillo (Arm), white; DAPI, blue. See also Supplementary Fig. 1 . ( c ′ –f ′) Schematics of cell organizations. Polar cells, red; presumptive border cells, green; gap cells, magenta asterisks. ( c , c ′) Radially symmetric organization of slbo -positive cells. ( d , d ′) Asymmetric organization of slbo -positive cells. ( e , e ′) One gap in slbo -positive cells around the polar cells. ( f , f ′) Two gaps in organization of slbo -positive cells. ( g ) STAT expression (red) is radially symmetric around the polar cells in seven neighbouring cells in wild type (WT; Canton S). (Arm, white.) ( h ) STAT activity (green) shows one gap around the polar cells, indicated by lack of 10XSTAT-GFP expression (white asterisk). (Arm, white.) ( i ) Seven Slbo-expressing cells (green) radially symmetric around the polar cells (yellow asterisks) in wild type. Apt, red, inset; Arm, white; DAPI, blue. ( j ) Two gaps (white asterisks) in slbo -reporter activation (green) next to the polar cells (yellow asterisks). Eyes absent (Eya), red, inset; E-cadherin (E-CAD), white; DAPI, blue. ( k ) Slbo protein (green) present in cells to one side of polar cells (yellow asterisks) (Fas III, white) and absent from two cells (white asterisks), although STAT (red, inset, arrows) is detected. ( l ) Proportions of four classes of organization patterns in the first tier of cells contacting the polar cells using four different markers/genotypes (bottom). For slbo reporter and 10XSTAT-GFP, positive cells were scored by GFP antibody staining. Numbers of egg chambers scored ( n ) shown at the top. Full size image We found significant variation among the patterns of Slbo and STAT expressing cells in the anterior epithelium, creating striking asymmetry in specification of motile cells. Genetic analysis shows that this variation is affected by the levels of STAT activity. Because Upd is released into an often-irregular domain bounded by nurse cells, we postulate that the landscape of adjacent tissue influences local morphogen concentrations and thereby cell fates. Simulations from our three-dimensional (3D) mathematical model of Upd dynamics and STAT activation in this cellular context support our hypothesis. Examination of mutant egg chambers with altered nurse cell arrangements and subapical architecture further indicates that cellular landscape influences morphogen distribution and adjacent cell fates. While the egg chamber provides a simple case, this work has broad implications in understanding the effects of diffusible signalling molecules more generally. Upright imaging reveals multiple patterns of cell activation Developing egg chambers are connected in ovarioles and are oblong, so they are generally viewed lying on their lateral side, obscuring cell fate patterning at the poles. Thus, the early organization of the border cells around the polar cells has not been clearly shown. During stage 8 of oogenesis, presumptive border cells arise near the polar cells in response to secreted Upd. Lateral views of egg chambers indicated that cells in contact with polar cells are fated to become migratory border cells, whereas those further away are fated as non-motile anterior follicle cells. This led to the conventional wisdom that the activated cells are arranged radially around the polar cells, and that all cells in contact with polar cells should be activated. To observe the pattern of border cell specification at the anterior, we developed a method to observe egg chambers end-on [24] . We first used the genotype slbo-Gal4, UAS-mCD8-GFP (referred to here as the slbo reporter; refs 25 , 26 and Fig. 1a ) to mark the border cells, which reveals the Slbo expression gradient across the anterior epithelium. We manually sorted and mounted individual egg chambers in glycerin jelly standing with the anterior end facing up (refs 24 , 27 and Fig. 1b ). We visualized horizontal cross-sections of vertical, late stage 8 egg chambers across multiple focal planes, revealing each cell of the anterior epithelium. When viewed upright, we expected every cell in contact with the polar cells to have activated STAT and also to express its target slbo . Interestingly, we found several different arrangements of presumptive border cells around the polar cells, assayed using the slbo -reporter line. In 25% of stage 8 egg chambers, slbo -positive cells formed a ring surrounding the polar cells in the expected radial pattern, and all cells contacting the polar cells were positive ( Fig. 1c and Supplementary Fig. 1 ). This configuration is consistent with the prediction that arises from postulating that Upd diffuses isotropically from a local source to activate JAK/STAT, and thus Slbo. Surprisingly, we found that a larger percentage of egg chambers (29%) revealed presumptive border cells all organized to one side of the polar cells ( Fig. 1d and Supplementary Fig. 1 ). In this case, only a few slbo -positive cells directly contacted the polar cells ( Fig. 1d ). This asymmetric pattern is contrary to what is expected if the polar cells release Upd and it diffuses evenly away, since follicle cells neighbouring the polar cells remained negative for slbo expression. We found a diversity of slbo -positive cell arrangements in the anterior epithelium. We grouped stage 8 egg chambers into four categories according to the activation pattern of the first tier of cells surrounding the polar cells: radially symmetric, asymmetric (activated to one side, both described above), one gap and two gaps or more ( Fig. 1c′–f′ ). The one gap class displayed one or two follicle cells in direct contact with the polar cells but not expressing slbo ( Fig. 1e ). The two or more gap arrangement was classified by appearance of two or more cells in contact with polar cells that did not express slbo , and did not contact each other ( Fig. 1f ). We only scored egg chambers with at least five positive cells to avoid younger stages, and because that was the smallest number of cells that could completely surround the polar cells. We observed similar total numbers of STAT-activated, slbo -positive cells in all arrangements, on average 6.5±0.6 s.e.m. ( Table 1 ). Notably, this is similar to the total number of follicle cells in direct contact with polar cells, which for this genotype was 6.5±0.2 s.e.m., and was consistent over different activation patterns ( Table 1 ). Thus, most arrangements of border cell precursors are not radially symmetric with respect to the polar cells. Table 1 Presumptive border cell number across organization. Full size table We used different markers to observe the specification patterns of border cells in detail. Examining STAT expression in wild-type (Canton S) egg chambers, or green fluorescent protein (GFP) expression in the STAT activity reporter line, 10XSTAT-GFP [28] , we found the same diversity in presumptive border cell arrangements as seen in the slbo -reporter line ( Fig. 1g,h,k,l ), and similar total numbers of positive cells ( Table 1 ). We also assayed egg chambers from a wild-type strain labelled with an antibody that detects Slbo protein. Again, we observed the same patterns of arrangements ( Fig. 1i–l ) and similar numbers of activated cells at stage 8 ( Table 1 ). We noticed some differences between the genotypes and markers, probably owing to slight differences in the timing of expression; from prior work [5] , we expect that STAT and its activity reporter would be activated first, followed by slbo reporter and then Slbo protein, which requires a high level of STAT activity (and therefore Upd) to be activated. It is also possible that the markers are differentially sensitive to detection, but we do not think this explains the different patterns observed because similar numbers of total presumptive border cells were detected in each case ( Table 1 ), and asymmetric patterns persisted into later stages ( Supplementary Fig. 2 ). Upon additional quantification, we found no significant difference between genotypes in the proportion of egg chambers exhibiting radial symmetry of Slbo-positive cells about the polar cells (using a χ 2 -contingency test, P value >0.05; Fig. 1l ). Using several markers, many egg chambers exhibited asymmetry of motile cell fate acquisition. In contrast, all anterior cells displayed expression of the STAT-negative regulator Apt ( Fig. 1i , inset), demonstrating that all cells are viable and equally visible by this imaging method. Follicle cell marker Eyes Absent (Eya) was also evenly expressed across the epithelium ( Fig. 1j , inset), further indicating that these anterior cells are all normal. Thus, surprisingly, some cells in contact with the polar cells fall below the STAT activity threshold necessary for border cell specification, demonstrated by the lack of nuclear STAT, STAT reporter expression or expression of the STAT target, Slbo. Raising STAT activity increases radial symmetry We considered several possibilities for how the asymmetry in presumptive border cell specification might occur. If too few cells became activated, this would generate asymmetry around the polar cells; however, contrary to this idea, we found in most genotypes 6–7 follicle cells contacted the polar cells, and in the majority of egg chambers at least this many presumptive border cells were activated ( Table 1 ). It was possible that one polar cell secreted much higher levels of Upd, however, this would result in the negative cells to be always oriented to one side of the polar cell pair, which was not the case (for example, Fig. 1d–f,j,k ). Another explanation for asymmetric activation of STAT around the polar cells could be intrinsic differences between cells of the epithelium, such as lack of Dome expression in some, or localized expression of an inhibitor. We did not observe obvious differences in dome-lacZ reporter expression across the anterior epithelium (refs 7 , 9 , 29 and Supplementary Fig. 3 ). To determine whether some follicle cells were refractory to STAT activation, we altered signalling levels. Genetic disruption of the negative regulator apt increases STAT activity in the anterior epithelium [19] . In upright egg chambers from flies homozygous for a loss-of-function mutation in apt ( apt KG05830 ), we saw significantly more Slbo-expressing cells at stage 8 than in controls (11.6±0.5 versus 6.1±0.7 s.e.m. ; P <0.0001 by ANOVA; Fig. 2a compare with Fig. 1f ), which is consistent with prior results. Most apt mutant egg chambers exhibited a radial organization of Slbo-expressing cells around the polar cells, a significant increase in this arrangement compared with controls ( Fig. 2a,f ; P <0.0001 in a χ 2 -contingency test). Almost all cells in contact with the polar cells were positive for Slbo and STAT in this genotype ( Fig. 2a,f and Supplementary Fig. 4 ). This demonstrates that all cells in this region are capable of STAT activation. 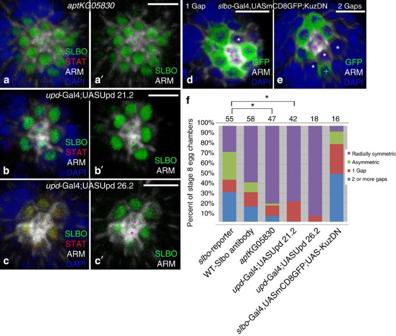Figure 2: Increased STAT activity increases radial symmetry in border cell specification. (a–e) Three-dimensional reconstructions of optical sections, projected into one plane, of anterior epithelia of mutant stage 8 egg chambers. Magenta asterisks indicate polar cells, whereas white asterisks indicate gap cells. Scale bars, 10 μm. (a–c) Slbo protein, green; STAT, red; Armadillo (Arm), white; 4,6-diamidino-2-phenylindole (DAPI), blue. See alsoSupplementary Fig. 4. (a) An egg chamber from anaptKG05830homozygote shows radial symmetry of Slbo-positive cells in the first tier of cells around the polar cells. (b,c) Overexpression of Upd in polar cells results in radial symmetry of Slbo-positive cells around the polar cells with either of two transgenes:upd-Gal4; UAS-Upd 21.2(b) orupd-Gal4; UAS-Upd 26.2(c). (d,e)slbo-Gal4, UAS-mCD8-GFP;UAS-KuzDNegg chambers display one (d) and two gaps (e) in border cell-specification patterns. GFP, green; Arm, white; DAPI, blue. The case ineis classified as two gaps because one gap cell touches the polar cells and a second is between the polar cells and a distantslbo-postive cell, indicated with a green +. (f) Proportions of four classes of arrangements of presumptive border cells at stage 8 for the following genotypes and markers:slbo-Gal4 reporter line (using GFP), wild type (Slbo antibody staining),aptKG05830(Slbo staining),upd-Gal4; UAS-Upd 21.2(Slbo staining),upd-Gal4; UAS-Upd 26.2 (Slbo staining),slbo-Gal4, UAS-mCD8-GFP;UAS-KuzDN(GFP antibody staining). Numbers of egg chambers scored are listed at the top of each column. A significant difference is indicated by *P<0.0001, in aχ2-contingency test. Figure 2: Increased STAT activity increases radial symmetry in border cell specification. ( a–e ) Three-dimensional reconstructions of optical sections, projected into one plane, of anterior epithelia of mutant stage 8 egg chambers. Magenta asterisks indicate polar cells, whereas white asterisks indicate gap cells. Scale bars, 10 μm. ( a–c ) Slbo protein, green; STAT, red; Armadillo (Arm), white; 4,6-diamidino-2-phenylindole (DAPI), blue. See also Supplementary Fig. 4 . ( a ) An egg chamber from an apt KG05830 homozygote shows radial symmetry of Slbo-positive cells in the first tier of cells around the polar cells. ( b , c ) Overexpression of Upd in polar cells results in radial symmetry of Slbo-positive cells around the polar cells with either of two transgenes: upd- Gal4; UAS -Upd 21.2 ( b ) or upd- Gal4 ; UAS-Upd 26.2 ( c ). ( d , e ) slbo- Gal4, UAS -mCD8-GFP; UAS -Kuz DN egg chambers display one ( d ) and two gaps ( e ) in border cell-specification patterns. GFP, green; Arm, white; DAPI, blue. The case in e is classified as two gaps because one gap cell touches the polar cells and a second is between the polar cells and a distant slbo -postive cell, indicated with a green +. ( f ) Proportions of four classes of arrangements of presumptive border cells at stage 8 for the following genotypes and markers: slbo -Gal4 reporter line (using GFP), wild type (Slbo antibody staining), apt KG05830 (Slbo staining), upd- Gal4; UAS -Upd 21.2 (Slbo staining), upd- Gal4; UAS -Upd 26.2 ( Slbo staining), slbo- Gal4, UAS -mCD8-GFP; UAS -Kuz DN (GFP antibody staining). Numbers of egg chambers scored are listed at the top of each column. A significant difference is indicated by * P <0.0001, in a χ 2 -contingency test. Full size image Next, we raised STAT activity in follicle cells by increasing Upd expression [9] , [10] , [11] , [12] , [21] . In the anterior epithelium, upd transcripts localize to the apical side of the polar cells [14] , but there is no report of asymmetry of Upd in other axes. We overexpressed Upd in the polar cells using the upd-Gal4 driver and two different overexpression transgenes (UAS- Upd21.6 and UAS -Upd26.2 ; ref. 21 ). With higher extracellular Upd, egg chambers exhibited radial symmetry of STAT activation about the polar cells much more often than controls ( Fig. 2b,c,f and Supplementary Fig. 4 ). In this case, cells that normally display low levels of STAT activation showed higher activity, indicated by high expression of Slbo protein, and significantly more cells had Slbo expression than in controls (8.6±0.3 versus 6.1±0.7 s.e.m., P <0.001). These results imply that few, if any, of the anterior follicle cells are intrinsically refractory to STAT activation, and suggest that a different mechanism must explain the asymmetric specification of border cells. Asymmetry in activation does not require Notch signalling Delta-Notch signalling is generally known for creating cellular heterogeneity during development and is necessary for cell specification in Drosophila [6] , [8] , [30] , [31] . During early oogenesis, Notch signalling regulates polar and follicle cell differentiation [32] , [33] , [34] , [35] . The Kuzbanian (Kuz) metalloproteinase cleaves and activates Notch and is highly expressed in the border cells [36] , [37] . Kuz, Delta and Notch are all required for normal border cell migration [37] , [38] . Thus, we considered whether Notch signalling influenced the asymmetry of cell specification. We inhibited Notch in border cells by expressing dominant-negative Kuz (referred to as Kuz DN ) [39] during mid-oogenesis. We observed that all the STAT activation patterns seen in control egg chambers, including asymmetry, exist in Kuz DN mutants ( Fig. 2d–f ), and in similar proportions to controls (no significant difference between pattern distributions by χ 2 -contingency tests). Eighty-one percent of mutant stage 8 egg chambers exhibited at least one gap in activation around the polar cells ( Fig. 2f ). Kuz DN egg chambers had the same number of Slbo-positive cells as controls (average of 6.0 versus 5.8, respectively, not significantly different in a two sample t -test, P >0.05), illustrating little or no change in the STAT threshold in the anterior epithelium. Thus, Notch signalling is unlikely to be required for asymmetry, although we cannot rule out that there may be some contributions from this pathway. Underlying tissue architecture affects response to Upd Our experiments demonstrated that STAT activity levels influence the border cell-specification patterns observed ( Fig. 2a–c,f ). We hypothesized that the asymmetric STAT activation in the epithelium could be caused by an uneven distribution of the Upd signalling molecule owing to the irregular domain created by the contours of the underlying tissue. The single-layer follicular epithelium lies above a cluster of large nurse cells ( Fig. 1a,b , inset). Anterior polar cells secrete Upd extracellularly towards the nurse cells, which do not significantly express the Upd receptor Dome ( Supplementary Fig. 3 ). While the nurse cells are generally space filling, regions where two or more cells meet create small extracellular domains or clefts ( Fig. 1b inset). Thus, the edges of the nurse cells could influence how Upd is distributed in the subapical extracellular domain and received by epithelial cells. We used markers for nurse cell boundaries and anterior imaging to visualize the domain adjacent to the epithelium. We stained egg chambers with fluorescent phalloidin to mark membrane-associated cortical actin, which provided an estimate for the cell edges. Although the clefts created by nurse cells varied in size, they appeared widest close to the epithelium and narrowed quickly towards the interior of the egg chamber ( Fig. 3a,b ), and tended to be smaller than a follicle cell. These subapical regions were roughly triangular in cross-section, and measured 10.7 μm 2 on average in the focal plane of polar cells when analysed in laterally imaged egg chambers ( n =14; Fig. 3a–b′ and Supplementary Table 1 , and see Methods section). We observed similar size clefts in upright 3D reconstructions ( Supplementary Movie 1 ). Although we observed several different arrangements, in 11% of wild-type egg chambers, one nurse cell juxtaposed the epithelium near the polar cells. More commonly (38% of cases), three nurse cells were positioned adjacent to the anterior-most follicular epithelium (assayed by nurse cell nuclei in the slbo -reporter genotype, n =38). We analysed in more detail the simple situation when the polar cells sat directly over a single nurse cell. In 4/7 of these cases, the STAT activation pattern was radially symmetric (for example, Fig. 3c–c′′′ , Supplementary Fig. 5 , Supplementary Movie 1 and Supplementary Table 2 ), consistent with Upd being relatively evenly distributed. However, in 3/7 of these egg chambers, some presumptive border cells sat over or near a cleft, and a gap in STAT activity was observed ( Supplementary Table 2 ). More complexity in patterns arose when more than 1 nurse cell lay in the anterior-most region of the egg chamber. When polar cell position aligned near a cleft created by two nurse cells, the STAT activation pattern had gaps and asymmetries ( Fig. 3d– e′′′ , and Supplementary Movies 2 and 3 ). In multiple cases, follicle cells over prominent clefts showed no activation ( Fig. 3e′′′ ), which might be expected if the extracellular domain acted as a sink for Upd. However, in some cases, follicle cells over clefts created by nurse cells did show activation, even if they were several cell diameters from the polar cells ( Fig. 3d′′′ and Supplementary Movie 2 ). How Upd might create this pattern was less clear. We were unable to examine Upd protein directly, as a fluorescently tagged reporter was not bright enough in vivo , and examination of extracellular protein in fixed tissue would not reveal signals where there are gaps between cells. Thus, to address our hypothesis, we developed a mathematical model. 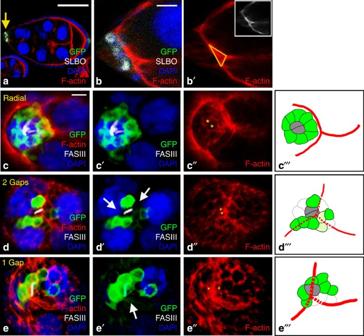Figure 3: Cell-specification patterns relative to adjacent nurse cell positions. (a–e) Staining for F-actin (with phalloidin, red) shows cell contours in stage 8slboreporter line egg chambers. (a) Wild-type egg chamber viewed laterally shows presumptive border cells at the anterior marked by Slbo expression (white, yellow arrow) and GFP (green). Scale bar, 50 μm. (b,b′) Magnified view of the anterior of the egg chamber shown ina; a subapical cleft created by the nurse cells can be seen adjacent to the activated cells. Scale bar, 10 μm. Yellow triangle inb′ shows the region measured to approximate the cleft dimensions (width along the apical side of the epithelium, depth from epithelium to where nurse cells meet). Inset shows F-actin staining alone. (c–c′′,d–d′′,e–e′′) Projections of optical sections from the anterior of egg chambers, including epithelium and top of underlying nurse cells. White arrows indicate gap cells. Yellow asterisks indicate polar cells.slboreporter, GFP, green; F-actin, red; Fasciclin III (Fas III), white; 4,6-diamidino-2-phenylindole (DAPI), blue. Scale bar is 7 μm. (c′′′,d′′′,e′′′) Schematics of presumptive border cell organization in the anterior epithelium. Polar cells are grey, presumptive border cells are green, presumptive border cells with low GFP expression are light green, gap cells are outlined in light grey, and the nurse cell cleft is red. Dotted portion of the cleft indicates the portion underlying anterior follicle cells. (c–c′′′) Radially symmetric organization ofslbo-positive cells. Polar cells and presumptive border cells positioned above nurse cell nuclei, with Y-shaped cleft to the right (see alsoSupplementary Fig. 5). (d–d′′′) Two gaps in organization ofslbo-positive cells around the polar cells. Polar cells positioned above the nurse cell cleft; arrows indicate gap cells touching polar cells. (e–e′′′) One gap organization ofslbo-positive cells around the polar cells. Polar cells positioned near the nurse cell cleft; arrow indicates gap cell region. See alsoSupplementary Movies 1–3. Figure 3: Cell-specification patterns relative to adjacent nurse cell positions. ( a – e ) Staining for F-actin (with phalloidin, red) shows cell contours in stage 8 slbo reporter line egg chambers. ( a ) Wild-type egg chamber viewed laterally shows presumptive border cells at the anterior marked by Slbo expression (white, yellow arrow) and GFP (green). Scale bar, 50 μm. ( b , b ′) Magnified view of the anterior of the egg chamber shown in a ; a subapical cleft created by the nurse cells can be seen adjacent to the activated cells. Scale bar, 10 μm. Yellow triangle in b ′ shows the region measured to approximate the cleft dimensions (width along the apical side of the epithelium, depth from epithelium to where nurse cells meet). Inset shows F-actin staining alone. ( c–c ′′, d–d ′′, e–e ′′) Projections of optical sections from the anterior of egg chambers, including epithelium and top of underlying nurse cells. White arrows indicate gap cells. Yellow asterisks indicate polar cells. slbo reporter, GFP, green; F-actin, red; Fasciclin III (Fas III), white; 4,6-diamidino-2-phenylindole (DAPI), blue. Scale bar is 7 μm. ( c ′′′, d ′′′, e ′′′) Schematics of presumptive border cell organization in the anterior epithelium. Polar cells are grey, presumptive border cells are green, presumptive border cells with low GFP expression are light green, gap cells are outlined in light grey, and the nurse cell cleft is red. Dotted portion of the cleft indicates the portion underlying anterior follicle cells. ( c–c ′′′) Radially symmetric organization of slbo -positive cells. Polar cells and presumptive border cells positioned above nurse cell nuclei, with Y-shaped cleft to the right (see also Supplementary Fig. 5 ). ( d–d ′′′) Two gaps in organization of slbo -positive cells around the polar cells. Polar cells positioned above the nurse cell cleft; arrows indicate gap cells touching polar cells. ( e–e ′′′) One gap organization of slbo -positive cells around the polar cells. Polar cells positioned near the nurse cell cleft; arrow indicates gap cell region. See also Supplementary Movies 1–3 . Full size image A computational model explains asymmetric Upd distribution To model Upd distribution in the 3D extracellular space, we used a partial differential equation that accounts for the change in Upd concentration over time due to the secretion, diffusion and uptake rates of this activator: for outward normal vector, n , where D represents the diffusion coefficient ( D =1 μm 2 s −1 ; which is within the range of diffusion coefficients determined for similar-sized molecules in Drosophila , as in refs 40 , 41 ). We estimated that Upd is released from the apical side of both polar cells at a rate of σ ( σ =45 pM μm s −1 , see Methods section), diffuses and is taken up by all follicle cells at the rate – ku with uptake proportionality constant k ( k =1 × 10 −4 s −1 ). (Since nurse cells had undetectable expression of the Upd receptor, we did not include uptake along this surface.) The source term was determined as the value necessary to achieve a threshold concentration of 3,900 pM, based on cell culture experiments [42] , and the uptake proportionality constant was converted to units of surface flux. We defined the domain of subapical extracellular space, Ω, ((−50 μm, 50 μm) × (−50 μm, 50 μm) × (0 μm, −0.2 μm)), that is bounded at the top by the apical surface of the epithelium, and at a distance, d , below by nurse cells ( Fig. 4a,b , see Methods section), using no-flux boundary conditions outside of the polar and follicle cells. In the base case, d =0.2 μm. We estimate a follicle cell surface size to be 5 μm × 5 μm. We refer to the space created by two juxtaposed nurse cells as the ‘cleft’ (length × width × depth). We considered cases in which one, two or three nurse cells were adjacent to the epithelium, and varied cleft dimensions accordingly. A 3D spatio–temporal simulation was then performed to estimate the concentration of Upd at all points in the domain. 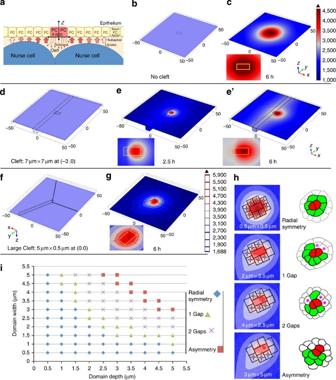Figure 4: Nurse cell landscape alters STAT signalling levels and cell-specification patterns. (a) Diagram shows follicle cells (FCs, yellow), polar cells (PCs, red), and adjacent nurse cells (blue), which create a cleft in the extracellular space (exaggerated for clarity). Domain coordinates are set to (0,0,0) at the apical point between PCs. PCs secrete Upd (dashed arrows). Upd uptake depends on its local concentration; darker red arrows indicate more uptake, whereas lighter arrows indicate less uptake. (b,d,f) Representations of the domain at the apical surface of the epithelium spanning 50 μm from the centre (PCs, rectangle). (b) A flat domain with no cleft. (c,e,e′) Heat maps show resultant Upd concentrations at the cell apical surface after simulations. Colour scale bar (to the right ofc) shows highest [Upd] in dark red; lowest in blue; insets magnify the flattened region around the PCs (yellow rectangle). (c) After a 6 h simulation, [Upd] is highest radially around the PCs and decreases with increasing distance. (d) A domain used forehas a rectangular region below one PC to approximate the cleft between two, subepithelial nurse cells, as ina. (e) Early, [Upd] is high to one side of the PCs and low above the cleft. (e′) Later, near-threshold levels of [Upd] (grey/pink) appear above the cleft. (f) A Y-shaped region centred at (0,0,0) approximates the cleft formed between three nurse cells, shown from the apical side for clarity (axes indicated). The variable-branch domain (left) of the cleft is sized at 5 μm deep × 0.5 μm wide, and the two constant branches at 0.5 μm × 0.5 μm. (g) Simulation using the domain fromfdepicts high [Upd] along the deepest cleft branch (colour scale to the right). (h) Simulations using domains with Y-shaped clefts yield the patterns of border cell specification observedin vivo(variable-branch size indicated). Cells approximated as 5 μm by 5 μm; diamonds indicate above-threshold [Upd] (presumptive border cells); scale as ing. Schematics as inFig. 1. (i) Different dimensions of the variable branch of a Y-shaped cleft determine different cell-specification patterns via simulations. Regions of the graph lacking points represent sizes for which no activation occurs. Figure 4: Nurse cell landscape alters STAT signalling levels and cell-specification patterns. ( a ) Diagram shows follicle cells (FCs, yellow), polar cells (PCs, red), and adjacent nurse cells (blue), which create a cleft in the extracellular space (exaggerated for clarity). Domain coordinates are set to (0,0,0) at the apical point between PCs. PCs secrete Upd (dashed arrows). Upd uptake depends on its local concentration; darker red arrows indicate more uptake, whereas lighter arrows indicate less uptake. ( b , d , f ) Representations of the domain at the apical surface of the epithelium spanning 50 μm from the centre (PCs, rectangle). ( b ) A flat domain with no cleft. ( c , e , e ′) Heat maps show resultant Upd concentrations at the cell apical surface after simulations. Colour scale bar (to the right of c ) shows highest [Upd] in dark red; lowest in blue; insets magnify the flattened region around the PCs (yellow rectangle). ( c ) After a 6 h simulation, [Upd] is highest radially around the PCs and decreases with increasing distance. ( d ) A domain used for e has a rectangular region below one PC to approximate the cleft between two, subepithelial nurse cells, as in a . ( e ) Early, [Upd] is high to one side of the PCs and low above the cleft. ( e ′) Later, near-threshold levels of [Upd] (grey/pink) appear above the cleft. ( f ) A Y-shaped region centred at (0,0,0) approximates the cleft formed between three nurse cells, shown from the apical side for clarity (axes indicated). The variable-branch domain (left) of the cleft is sized at 5 μm deep × 0.5 μm wide, and the two constant branches at 0.5 μm × 0.5 μm. ( g ) Simulation using the domain from f depicts high [Upd] along the deepest cleft branch (colour scale to the right). ( h ) Simulations using domains with Y-shaped clefts yield the patterns of border cell specification observed in vivo (variable-branch size indicated). Cells approximated as 5 μm by 5 μm; diamonds indicate above-threshold [Upd] (presumptive border cells); scale as in g . Schematics as in Fig. 1 . ( i ) Different dimensions of the variable branch of a Y-shaped cleft determine different cell-specification patterns via simulations. Regions of the graph lacking points represent sizes for which no activation occurs. Full size image The computational model was run for different lengths of time and a range of hypothetical source terms to see the effects on morphogen distribution over time. We set Upd concentration to 0 pM at time zero, and set a threshold level of 3,900 pM for the concentration sufficient to activate and maintain STAT signalling, as this is consistent with physiological levels in cell culture [42] . We generated contour plots to determine the morphogen concentration at the apical epithelial boundary (where z =0 μm in the domain; Fig. 4a ). As expected, when modelled with an even underlying domain (no cleft; Fig. 4b ), Upd signal at a concentration higher than 3,900 pM arose in a radially uniform ring around the polar cells ( Fig. 4c ), which would activate STAT in surrounding cells. Since the model is linear up to the source term, increasing σ increases the concentration at the epithelial surface (and increases the likelihood of activating more cells, as in Upd overexpression; Fig. 2 , and see below). Increasing D would increase the spread of Upd in the same amount of time, and increasing k would decrease the spread of Upd by increasing the uptake. As a first test, we also explored the outcome when only one polar cell secreted Upd ( Supplementary Fig. 6 ). As we expected, follicle cells nearest to the secretory polar cell became activated, whereas those to the other side were not ( Supplementary Fig. 6c ). However, there is no evidence one polar cell is inactive, and since our asymmetric patterns of activation in vivo did not consistently align to one side of the polar cell pair, this idea did not explain the majority of the asymmetries we observed. Next, we introduced different underlying cleft geometries into the computational model to see how this affected Upd distribution and cell activation. We began with a simple case: two nurse cells and one cleft under the polar cells ( Fig. 4d ). In this case, a 7 μm-wide cleft acted as a sink in short time frames (2.5 h), shifting high STAT activation to the other side of the polar cells only (indicated by the heat maps in Fig. 4e ), even though both cells secreted Upd. At longer times (6 h), a different asymmetry was observed: higher levels of Upd expanded along the cleft, potentially at high enough levels for border cell specification along that domain ( Fig. 4e′ ). This suggests that once Upd is released into the cleft, it fills up the ‘sink’ and then disperses into the surrounding area. At late times, this crevice behaves as a source of Upd, although at a lower level than the polar cells. We next replicated the common three nurse cell arrangement in the computational model to determine how this impacted Upd distribution. This organization of nurse cells leads to a Y-shaped crevice ( Fig. 4f,g ). In this case, we performed a parametric sweep by altering the dimensions of a single branch of the cleft to range between 0.5 and 5 μm in depth and width, respectively. This size range, because it is modelled as a rectangular prism domain, roughly maps to the volume of the concave triangular prism domains observed in egg chambers. Over this range, the computational model unexpectedly yielded all four cell-specification patterns observed in vivo ( Fig. 4h,i ). If we significantly increased the source term ( σ =75 pM μm s −1 ) to represent overexpression of Upd (as in Fig. 2 ), radial symmetry was restored even when including a Y-shaped cleft ( Supplementary Fig. 7 ). Thus, our model implies that underlying tissue contour alters how morphogens signal to adjacent tissue, and thereby modulates cell-specification patterns. Enlarged subapical domain results in symmetrical activation To test further the hypothesis that underlying tissue geometry influences morphogen distribution, we examined mutant egg chambers that had fewer nurse cells. Specifically, we used mutant alleles of the gene half pint ( hfp ; which encodes Poly U binding factor 68kD), in which nurse cells often fail to complete the correct number of cell divisions [43] , [44] . We confirmed that females bearing viable combinations of two different mutant alleles ( hfp 38 /hfp 13 ), or heterozygous mutant females for a strong allele ( hfp 13 /+), developed stage 8 egg chambers that had fewer than the normal 15 nurse cells, averaging 10.8 or 12.0, respectively ( Fig. 5a ; n =16). We did not detect any abnormalities in gross follicle cell development using these alleles ( Fig. 5b and Supplementary Fig. 8 ), which is consistent with prior reports that primarily germline cells are disrupted [43] . 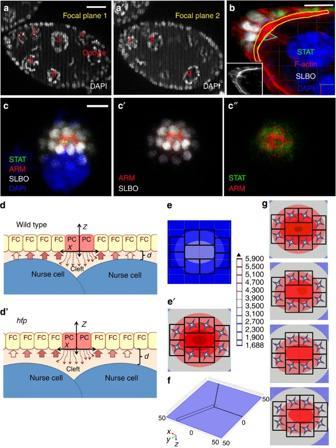Figure 5: Larger extracellular spaces and radially symmetric STAT activation inhfpmutants. (a, a′)hfp13/TM2mutant egg chambers contain fewer nurse cells. Nurse cell nuclei, DNA stained with 4,6-diamidino-2-phenylindole (DAPI), are numbered in two focal planes of one egg chamber. Scale bar, 20 μm. (b) A lateral view of the anterior epithelium and nurse cells in an egg chamber from ahfp38/hfp13female; phalloidin marks cortical actin (red); DAPI marks DNA (blue); STAT (green) and Slbo (white) expression is detected by antibodies. Nurse cells are not tightly packed against the epithelium, leaving an abnormally large extracellular space (domain outlined in yellow). The cleft domain between two nurse cells is relatively small (cyan outline). Inset shows F-actin staining alone. Scale bar, 10 μm. (c–c′′) Anterior of anhfp38/hfp13mutant egg chamber. All cells surrounding the polar cells (PCs; yellow asterisks, outlined by Armadillo (Arm) expression, red) have high STAT activation levels, reflected by Slbo (white,c′) and STAT (green,c′′) expression. In this egg chamber, only one nurse cell lies below the anterior epithelium, seen by DAPI staining. Scale bar, 10 μm. (d,d′) Schematics depict the wild-type subapical extracellular domain (d) and that inhfpmutants (d′), which is deeper (marked withd). (e,e′) Simulations to modelhfpmutants with deeper subapical domains (d=0.5 μm) and no cleft shows no activation whenσ=45 pM μm s−1(e), but a modest increase in source levels toσ=65 pM μm s−1results in radial activation of follicle cells (FCs) (e′), scale to right. (f) A Y-shaped domain with one variable cleft at the left. (g) Simulations to modelhfpmutants with deeper subapical domains (d) and Y-shaped clefts show radially symmetric activation about the PCs for all size variants (scale as ine). Variable-branch sizes: top panel: 0.5 μm wide × 0.5 μm deep, second panel: 2 × 3.5 μm, third panel: 4 × 2.5 μm and bottom panel: 3 × 5 μm. Figure 5: Larger extracellular spaces and radially symmetric STAT activation in hfp mutants. ( a, a ′) hfp 13 /TM2 mutant egg chambers contain fewer nurse cells. Nurse cell nuclei, DNA stained with 4,6-diamidino-2-phenylindole (DAPI), are numbered in two focal planes of one egg chamber. Scale bar, 20 μm. ( b ) A lateral view of the anterior epithelium and nurse cells in an egg chamber from a hfp 38 /hfp 13 female; phalloidin marks cortical actin (red); DAPI marks DNA (blue); STAT (green) and Slbo (white) expression is detected by antibodies. Nurse cells are not tightly packed against the epithelium, leaving an abnormally large extracellular space (domain outlined in yellow). The cleft domain between two nurse cells is relatively small (cyan outline). Inset shows F-actin staining alone. Scale bar, 10 μm. ( c–c ′′) Anterior of an hfp 38 /hfp 13 mutant egg chamber. All cells surrounding the polar cells (PCs; yellow asterisks, outlined by Armadillo (Arm) expression, red) have high STAT activation levels, reflected by Slbo (white, c ′) and STAT (green, c ′′) expression. In this egg chamber, only one nurse cell lies below the anterior epithelium, seen by DAPI staining. Scale bar, 10 μm. ( d , d ′) Schematics depict the wild-type subapical extracellular domain ( d ) and that in hfp mutants ( d ′), which is deeper (marked with d ). ( e , e ′) Simulations to model hfp mutants with deeper subapical domains ( d= 0.5 μm) and no cleft shows no activation when σ =45 pM μm s −1 ( e ), but a modest increase in source levels to σ =65 pM μm s −1 results in radial activation of follicle cells (FCs) ( e ′), scale to right. ( f ) A Y-shaped domain with one variable cleft at the left. ( g ) Simulations to model hfp mutants with deeper subapical domains ( d ) and Y-shaped clefts show radially symmetric activation about the PCs for all size variants (scale as in e ). Variable-branch sizes: top panel: 0.5 μm wide × 0.5 μm deep, second panel: 2 × 3.5 μm, third panel: 4 × 2.5 μm and bottom panel: 3 × 5 μm. Full size image Presumptive border cell activation patterns in hfp mutant egg chambers differed significantly from controls, with 100% of stage 8 egg chambers exhibiting radial organization of Slbo-expressing cells (compare Fig. 5c with Fig. 1c–f ). In 41% of egg chambers examined (7/16), only one nurse cell juxtaposed the anterior epithelium, and, as in the ‘no cleft’ case, all of the follicle cells contacting the polar cells were positive for markers of STAT activity, including Slbo and STAT proteins ( Fig. 5c ). Remaining egg chambers predominantly had 2–3 nurse cells at the anterior, but in these cases the nurse cells did not fill the space as completely as in wild type. As a result, a gap was created between the epithelium and the nurse cells ( Fig. 5b,d′ ), generating abnormally large subapical extracellular areas. We estimated this cross-sectional area by measuring a straight-edged crescent shape, excluding the relatively small region of the divot for simplicity (see Fig. 5b , in which the measured domain is outlined). Although this underestimates the total area, we still found the subapical domain in hfp mutants to be significantly larger than in controls, ranging 18–48 μm 2 in cross-section ( Fig. 5b and Supplementary Table 1 ). Interestingly, these cases showed normal numbers of presumptive border cells contacting the polar cells, and radially symmetric activation over a larger region, in spite of the large cleft(s) ( Table 2 ). Table 2 Presumptive border cell numbers and arrangements in half pint (hfp) loss-of-function mutant egg chambers. Full size table We next used these data to validate the computational model further. First, we tested the case for one nurse cell near the epithelium and a uniform subapical extracellular domain. As would be expected, with an increase in subapical space by 2.5 times (or 150%), we saw a decrease in signal strength resulting in no above-threshold cells in the model output ( Fig. 5d,e ). However, a modest (44%) boost in release strength from 45 to 65 pM μm s −1 results in radially symmetric activation, which is similar to the case for one nurse cell adjacent to the anterior follicle cells ( Fig. 5e′ ). Moreover, when we modelled this situation with irregular underlying domains, mimicking three nurse cells at the anterior, a similar number of cells were activated but in a radially symmetric pattern for all cleft cases, where one branch of the Y-shaped cleft is varied ( Fig. 5f,g ). This modelling result is consistent with the subapical spacing measured in the 2D view, and the increased symmetry in the activation pattern found experimentally in the hfp mutants with a smaller numbers of nurse cells. These results validate the computational model and further support the importance of the proximity of the nurse cells in guiding extracellular signalling. Previous studies suggested that the follicle cells closest to the polar cells receive the highest levels of Upd, maintain above-threshold STAT activity and therefore become fated as migratory [9] , [10] , [11] , [12] , [19] . This implies that proximity to the polar cells is critical to border cell specification. We find that contact with the polar cells is not sufficient to lead to border cell fate. Some follicle cells touching the polar cells do not achieve above-threshold levels of STAT activation. These ‘gap’ cells are of normal follicle cell lineage, indicated by the presence of Apt and Eya proteins, and are capable of receiving signal, as shown when we increased STAT signalling levels. We found no evidence of cell death assayed by activated caspase 3 (ref. 45 ) staining ( Supplementary Fig. 9 ), and the position of the unactivated cells varied in their alignment with the two polar cells. Differences in the patterns of GFP-marked cells and endogenous proteins in some cases (for example, Fig. 1k ), and discontinuities between GFP-positive cells (as in Figs 1h,j and 2e ) suggest that movement between follicle cell ring canals [46] is not sufficient to explain asymmetries either. Moreover, asymmetric border cell patterns persist into stage 9, which suggest that cell rearrangement is unlikely to cause the asymmetries ( Supplementary Fig. 2 ). We propose that the cells negative for Slbo expression at stage 9, but in contact with polar cells, dissociate from the border cell cluster and are fated to become stretch cells. We favour the hypothesis, supported by computational modelling, that some anterior follicle cells near polar cells are not exposed to high Upd concentrations because this signalling molecule is funnelled away by adjacent domains, resulting in asymmetries of STAT activation. Cells further from the polar cells may receive high Upd along adjacent, funnelling clefts, but at a later time. This is reminiscent of results in Zebrafish showing that collection of morphogen in pockets of tissue influences the responses of nearby cells [47] . When too few or too many border cells are specified, migration is disrupted, suggesting that there is an optimal number of motile cells, usually between 6–8 (ref. 5 ). It was postulated that the cells closest to the polar cells all became motile, which would limit the number of border cells, since, on average, 6.4 follicle cells can fit around the polar cells ( Table 1 ). Our results suggest, though, that a more complex counting mechanism must operate to ensure that a sufficient number of cells are specified: this system must be robust enough to buffer the effects of various possible distributions of the activating protein due to differences in the underlying tissue geometry. In addition, it is curious that even mutant egg chambers with large subapical extracellular domains can specify a large number of presumptive border cells. A compensatory mechanism to upregulate Upd or STAT signalling may exist to allow sufficient signalling in this case. Our mathematical model demonstrates that the underlying tissue on the apical side of the anterior epithelium is sufficient to alter the spatial distribution of Upd, and thereby explain the asymmetric specification of border cells. Interestingly, our model suggests that the impact of a cleft on local concentrations of signalling molecules changes with time: earlier it may act as a sink for a secreted factor, whereas later the factor is pooled along the cleft, thereby increasing its available levels for signalling to the adjacent tissue. Currently, it is difficult to observe the position of the cleft relative to the border cells and the precise size of the domain, and these may shift as the egg chamber develops. Thus, it is not surprising that we did not see exact alignment of clefts and activated cells, since Upd distribution and cell surface binding occurs hours before we examined the cell activation patterns. However, the model recapitulates the in vivo specification patterns over a wide range of cleft sizes and positions, and even small clefts had a detectable impact. While the development of this model took advantage of the relatively simple tissue architecture of the Drosophila egg chamber, it is likely to be relevant in other contexts [48] and could be adapted. Little research has investigated the role of extracellular domains on the actions of diffusible signalling molecules, although several studies have considered three dimensions more generally, or how cell packing creates ‘tortuosity’ in the domains morphogens traverse [1] , [3] , [47] , [48] . Developing leg and wing imaginal discs, though, have epithelial sheets of complex topography that bound the domains in which morphogens act [49] , [50] , so this may provide a comparable situation. For tissues in which cells are very tightly packed, secreted signals must move through complex paths. In vertebrate developing limbs, the effects of signalling molecules such as retinoic acid, fibroblast growth factors (FGFs) and Sonic hedgehog are likely to be altered by how they diffuse between cells, which is considered in some models [51] , [52] . Similarly, in the mammalian brain, how tightly cells are arranged has been shown to affect the distribution of signalling molecules, even when there are only small gaps between cells [53] , [54] . Notably, recent studies demonstrate that FGF can pool in microluminal domains to concentrate its effect in Zebrafish lateral line migration [47] . Thus, our work strongly supports the idea that to understand how diffusible signalling molecules control cellular responses, the influence of the surrounding complex landscape must be taken into consideration, and that modelling will improve our understanding of these effects. Drosophila genetics Fly stocks and crosses were maintained at 25 °C. Flies were incubated at 29 °C for 16 h before dissection for optimal Gal4/UAS transgene expression. The following genotypes were used: Canton S (wild type, Bloomington Stock Center); slbo reporter= slbo -Gal4 (ref. 25 ), UAS-mCD8-GFP/CyO (ref. 26 ); STAT activity reporter=10XSTAT92E-GFP (ref. 28 ); UAS- Kuz DN (ref. 39 ) (Bloomington Stock Center); enhancer trap upd -Gal4, UAS- Upd 21.2 and UAS- Upd 26.2 (ref. 21 ; provided by Dr D. Montell); apt KG05830 insertional mutant stock [19] , [55] (Bloomington Stock Center); hfp 9 , th, st, cu, sr, e/TM2; hfp 13 , st, cu, e, ca/TM2, Ubx and hfp 38 , st, cu, e, rec2/TM2 stocks [43] (gifts from Dr G. Schüpbach); dome -LacZ= w 67c23 P{lacW} dome G0282 /FM7c (Bloomington Stock Center). Immunofluorescence Ovary dissection and staining was performed using standard methods [56] . Briefly, fixation was performed using 4% formaldehyde in 0.1 M phosphate buffer (pH 7.4) for 10 min. After washing in NP40 buffer, the following primary antibodies and dilutions were used in overnight incubation: rat anti-Drosophila E-cadherin (1:25; ref. 57 ), mouse anti-Fasciclin III (Fas III; 1:50; ref. 58 ), mouse anti-Armadillo (anti-Arm; 1:40; ref. 59 ), mouse anti-Eya 1 (1:1,000; ref. 60 , DCAD2, Fas III 7G10, Arm N2 7A1 and Eya 10H6 antibodies from the Developmental Studies Hybridoma Bank, developed under the auspices of the NICHD, and maintained by the University of Iowa, Department of Biology, Iowa City, Iowa 52242); rat anti-Slbo (1:1,000; ref. 11 ), rabbit anti-STAT (1:1,000; ref. 61 ) and rabbit anti-APT (1:1,000; ref. 64 ) were gifts from Drs P. Rorth, D. Montell, and R. Schuh, respectively. For Supplementary Figs , the following additional primary antibodies and dilutions were used: chicken anti-β-galactosidase (1:500, Aves) and rabbit anti-cleaved caspase 3 (1:400, Cell Signaling). After washes, the following secondary antibodies and dilutions were used: chicken anti-GFP (1:250; Life Sciences), Molecular probes Alexa Fluor secondary antibodies (488, 568 and 647 nm; 1:400). 4,6-diamidino-2-phenylindole (DAPI; 1:1,000; Life Sciences) was added for 10 min after secondary antibodies, then washed out. To visualize cortical actin in the nurse cells, Alexa-568-Phalloidin dye was added to egg chambers (1:50; Life Technologies) in 1 × PBS (Sigma-Aldrich) with 1% bovine serum albumin (VWR) and incubated for 25 min, followed by several washes in NP40 buffer. Upright imaging Upright imaging method is described in detail in ref. 24 . Briefly, melted glycerin jelly was spread over microscope slides and chilled overnight. Stage 8 or 9 egg chambers were chosen under a Leica fluorescent stereoscope, transferred with a needle to the slides, and covered with glycerine jelly and chilled at 4 °C overnight. Columns of mounted egg chambers were cut out under a dissection scope using 45° angle miniature scalpel (Fine Science Tools) and transferred to a coverslip with anterior side of egg chambers facing down. Coverslips and blocks were mounted on slides and imaged upright. Upright images were acquired on a Leica SP5 confocal microscope equipped with Leica LAS software. Three-dimensional reconstructions of upright egg chamber optical sections were acquired using PerkinElmer Volocity 3D Image Analysis software, which allows volumetric analysis and projections of stacks of images into 2D representations. Upright imaging experiments were performed at least three times for each genotype, and data were pooled. Horizontal images were acquired on a Zeiss Axioimager Z1 microscope equipped with Axiovision software and the Apotome structural interference system (Zeiss) for optical sectioning. Adobe Photoshop CS6 was used to process and format images. For cell counts, both 3D projections and Z-stacks of individual optical sections were analysed, both as single channels and in overlays, to identify individual cells. Optical sections were acquired from the first focal plane that displayed signal through the extent of border cell marker expression. Depth and width of clefts identified by 3D projections were measured in laterally mounted egg chambers using Leica LAS software, and using cortical actin to approximate the cell surface. Cleft depth was measured from the apical border of polar cells to the deepest part of a V created by edges of two adjacent nurse cells, in μm; clefts were only considered if the V lay directly adjacent to activated cells; cleft width was measured from the apex of the nurse cell (the part closest to the follicular epithelium) to the apex of the neighbouring nurse cell. Cleft area was determined by the approximation 1/2 × width × depth. Measurements were consistent between lateral and upright egg chambers. Upright egg chambers were analysed using Volocity Imaging Software to rotate image planes. Mathematical modelling We created a 3D representation of the extracellular domain between epithelium and nurse cells using COMSOL Multiphysics (Comsol Multiphysics 3.5a), a finite element analysis software, and used COMSOL’s general form PDE module to create simulations of the time-dependent diffusion of Upd using the equations shown in the text. The domain was constructed of two contiguous components: a thin space between epithelium and nurse cells Ω ((−50 μm, 50 μm) × (−50 μm, 50 μm) × (0 μm, −0.2 μm)) and a cleft between nurse cells. The cleft is either a single gap between two nurse cells ((−50 μm, 50 μm) × cleft width × cleft depth) or a Y-shaped gap between three nurse cells, with one of the three branches modelled as a variable cross-section (cleft width × cleft depth), and the other two as constant cross-sections (0.5 μm × 0.5 μm). Clefts were modelled as rectangular prisms, since our analyses showed that the area of the domain, not its shape, was the feature that gave rise to changes in activation. The Upd source, via secretion from the polar cells, was positioned at the centre of the epithelial surface with uptake along the top surface, excluding the polar cells, and zero flux at the nurse cell boundaries, and imposed domain ends. We derived the essential influx of Upd (45 pM μm s −1 ) to elicit a concentration in the range of 4,000 pM at about the 6 h mark in line with in vitro experiments [42] . (We can also confirm that this value for sigma is reasonable by estimating a vesicular density times vesicular release rate to yield: where the vesicle density of Upd, which is ∼ 10 times larger than insulin, would take about a factor of 1,000 fewer molecules per vesicle (ref. 62 ) (5 × 10 5 with a release rate reasonably lower than that of insulin (1 μm −2 s −1 ; ref. 63 . The maximal decay rate (5 × 10 −4 s −1 ) in a volume given in ref. 37 is transformed into the surface uptake flux by imposing the surface to volume ratio in the thin epithelium-nurse cell space, 0.2 μm, to get k =1 × 10 −4 s −1 .) The diffusion coefficient is a middling estimate from refs 41 , 40 . The distance between the epithelium and nurse cells in wild type was d =0.2 μm, cleft geometries were constructed using blocks of variable dimension, and the depth and width of the blocks were modified using parametric sweeps. In order to imitate the top–down perspective visualized in fluorescent imaging, our solution set was graphically analysed in a volume plot with overlaid contours and a multislice grid. Each square on the grid represented an individual follicle cell, and cells that received a concentration above 3,900 pM over 50% of their surface were determined to be activated for border cell specification and motility. Colour scales for the heat maps shown in Figs 4 and 5 , and Supplementary Figs 6 and 7 show middle range values to allow comparisons. We were able to compare our upright imaging views of border cell activation patterns to those predicted by the COMSOL 3D plot groups. How to cite this article: Manning, L. et al. Tissue landscape alters adjacent cell fates during Drosophila egg development. Nat. Commun. 6:7356 doi: 10.1038/ncomms8356 (2015).